Magnetic switching of ferroelectric domains at room temperature in multiferroic PZTFT Single-phase magnetoelectric multiferroics are ferroelectric materials that display some form of magnetism. In addition, magnetic and ferroelectric order parameters are not independent of one another. Thus, the application of either an electric or magnetic field simultaneously alters both the electrical dipole configuration and the magnetic state of the material. The technological possibilities that could arise from magnetoelectric multiferroics are considerable and a range of functional devices has already been envisioned. Realising these devices, however, requires coupling effects to be significant and to occur at room temperature. Although such characteristics can be created in piezoelectric-magnetostrictive composites, to date they have only been weakly evident in single-phase multiferroics. Here in a newly discovered room temperature multiferroic, we demonstrate significant room temperature coupling by monitoring changes in ferroelectric domain patterns induced by magnetic fields. An order of magnitude estimate of the effective coupling coefficient suggests a value of ~1 × 10 −7 sm −1 . The search for room temperature magnetoelectric multiferroics is driven by a strong desire to fabricate novel functional devices [1] , [2] , [3] : tunnel junctions that can be controlled electrically, rather than magnetically, for example, or new non-volatile memories that can be written electrically, but read magnetically. It is envisaged that such devices would combine the advantages of both ferroelectricity and ferromagnetism; a multiferroic memory is a good illustration of this, as the sub-nanosecond switching speeds and ultra-low power voltage-driven WRITE operations, associated with ferroelectric random access memory, could be combined with the non-destructive READ operations, characteristic of magnetic random access memory. A detailed discussion of potential applications can be found in the recent review by Pyatakov and Zvezdin [2] . For the majority of such proposed devices, two material characteristics are vital: first, that multiferroic behaviour occurs at room temperature and second, that there is significant coupling between ferroelectric and magnetic properties. Achieving both of these characteristics in a single material has so far been a major challenge for research: TbMnO 3 (ref. 4 ), TbMn 2 O 5 (ref. 5 ) and YMnO 3 (refs [6] , [7] 6,7) are well established systems, but only display multiferroicity at cryogenic temperatures; recently CuO has also been shown to possess multiferroicity [8] , [9] , but again only significantly below room temperature (230 K) and, even when cooled, it possesses a small electrical polarization, which is perhaps not surprising given that it is the magnetic ordering that induces the ferroelectricity [9] ; EuTiO 3 thin films, grown on mismatched substrates, which induce biaxial tension, represent a remarkable discovery, and another landmark for strain-engineering [10] , but again are not multiferroic at room temperature. Doped ZnO has been claimed as a room temperature multiferroic [11] , [12] , but ferroelectricity in ZnO, first reported in 1996 [13] , is highly contentious. Strong symmetry arguments point towards electret rather than true ferroelectric behaviour. Sr 3 Co 2 Fe 24 O 41 (ref. 14 ) could operate at room temperature, and unlike most magnetoelectrics does not require a prohibitively high (order of a Tesla) magnetic field to switch [14] ; it does, however, require a magnetic bias field and hence cannot be a bilinear magnetoelectric. Other interesting work has seen spiral magnetic ordering inducing a ferroelectric phase transition [15] , but again room temperature operation is a major challenge. Multiferroic heterostructures, which demonstrate magnetoelectric behaviour through various modes of interlayer coupling (strain-mediated, exchange bias mediated or charge-coupling mediated) [16] , are a serious alternative to single-phase materials and have been demonstrated to have obvious potential [16] , [17] , [18] , [19] , [20] , [21] , [22] , [23] : full room temperature magnetisation reversal, by application of an electric field, has been realized by Heron et al . [22] and recently the ability to precisely write ferromagnetic domains with a low electric field was shown by Lahtinen et al . [23] —a remarkable achievement for spintronic devices. The largest coupling coefficient in any system of which we are aware is 10 −6 sm −1 in CoFe-BaTiO 3 heterostructures [23] . A more complete summary of work to date, focusing on magnetoelectric heterostructures, can be found in the recent review by C A F Vaz [16] . Surprisingly, until very recently [24] , [25] , the only single-phase material to demonstrate both unambiguous room temperature multiferroicity and magnetoelectric coupling was BiFeO 3 (ref. 25 ). Unsurprisingly, it has become the most studied of all multiferroic materials [27] . The renaissance of interest in BiFeO 3 was largely because of the successful growth of epitaxial thin films (initially by Ramesh and coworkers) that demonstrated ferroelectric polarisation values of the order of 100 μC cm −2 , and saturation magnetization of 150 emu cm −3 (refs 2 , 28 ). Thin films have not only been studied as single layer multiferroics, but have also been highly successfully integrated into magnetoelectric heterostructures [19] , [22] , [29] . However, even BiFeO 3 is far from the ideal multiferroic: the prospects of realising useful devices might be limited by high electrical conduction [30] and by complications associated with a plethora of phase transitions [30] , both in surface layers and within the bulk. The discovery of an alternative room temperature multiferroic material, by several of the authors, is therefore potentially highly exciting. Solid solution phases between lead zirconium titanate (PZT) and lead iron tantalate (PFT) end member perovskites [24] (PZTFT) have demonstrated both ferroelectric and ferromagnetic/ferrimagnetic hysteresis loops at room temperature. This might seem surprising, given that PbFe 1/2 Ta 1/2 O 3 (like PbFe 1/2 Nb 1/2 O 3 (ref. 31 )) possesses a Néel temperature around 150 K, and shows magnetic susceptibility characteristics of an antiferromagnet. Even it, however, shows ‘ferromagnetic’ hysteresis loops up to 300 K or above due to spin clustering. Crucially, in PZTFT solid solution materials, polarization-electric field hysteresis curves have been found to change, slightly but demonstrably, under applied magnetic fields [24] . Given the subtle nature of this apparent magnetoelectricity, further research to make more explicit statements on coupling behaviour have become an imperative in order to gauge the importance of this new material for potential device applications. In this article, we have used piezoresponse force microscopy (PFM) imaging of single-crystal slices or lamellae of PZTFT to demonstrate an unequivocal change in ferroelectric domain patterns induced by the application of a magnetic field at room temperature. Large changes in ferroelectric domain states were found to be stochastic and unpredictable. However, more modest ferroelectric domain changes were found to be more reproducible and controllable and could be reversed to some extent by changing the orientation of the applied magnetic field. The study echoes seminal work done at cryogenic temperatures on MnWO 4 using second harmonic imaging techniques [31] . Characterization of microstructure Initial characterization of the single-crystal slices ( Fig. 1 ), using transmission electron microscopy (TEM) techniques, showed that even within a single-crystal lamella (cut from a single grain in a coarse grained ceramic—see Methods) the microstructure is extremely rich. Domains, with curved domain walls, are present both as individual units and grouped into bundles, such that structure occurs across a number of different length scales. When selected area diffraction patterns were taken across different regions, they were extremely similar ( Fig. 1b ) strongly suggesting that domain variants had formed from a single higher symmetry parent state. A series of points was sampled, using energy dispersive X-ray (EDX) spectroscopy, to determine both cation chemistry and to gauge chemical homogeneity. No obvious heterogeneity was apparent within the single-crystal lamellae, but the cation composition was found to differ slightly from the intended [Pb(Zr 0.53 Ti 0.47 )O 3 ] 0.6 —[Pb(Fe 0.5 Ta 0.5 )O 3 ] 0.4 . Measured cation content was PbZr 0.296±0.004 Ti 0.168±0.004 Fe 0.174±0.002 Ta 0.272±0.008 , where uncertainties are given by the standard error across all the EDX measurements taken. 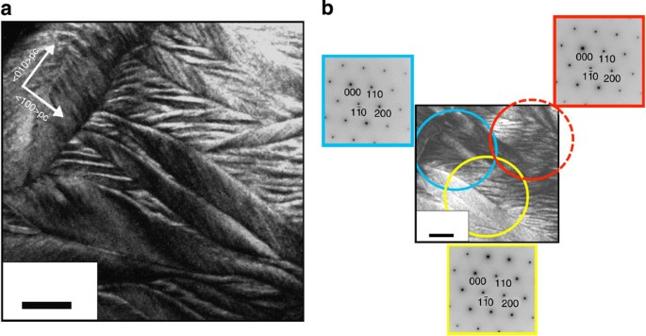Figure 1: Complex domain structures in PZTFT single crystal. Scanning transmission electron microscopy (STEM) reveals a rich microstructure in which domains form into irregular patterns, with domain walls that do not obviously adhere to strict crystallographic orientations (a). Despite this complexity, it seems that all the domain variants have formed from a single higher symmetry parent state, as the selected area diffraction patterns from different regions, indicated by the coloured circles in (b), are indistinguishable. Scale bar, 200 nm. Figure 1: Complex domain structures in PZTFT single crystal. Scanning transmission electron microscopy (STEM) reveals a rich microstructure in which domains form into irregular patterns, with domain walls that do not obviously adhere to strict crystallographic orientations ( a ). Despite this complexity, it seems that all the domain variants have formed from a single higher symmetry parent state, as the selected area diffraction patterns from different regions, indicated by the coloured circles in ( b ), are indistinguishable. Scale bar, 200 nm. Full size image Domain microstructure was also imaged using PFM. Left and middle panels in Fig. 2a illustrate typical amplitude images from lateral-mode PFM (see Methods ). Piezoelectrically active domains are clearly evident and both domains and bundles of domains can again be observed. Although, in general, the observation of a domain hierarchy is commensurate with the TEM/scanning transmission electron microscopy (STEM) imaging, we note the different length scales involved in Figs 1 , 2 . The fine stripe contrast resolved under PFM correlates with the domain bundles imaged under TEM/STEM. It therefore appears that there are at least three levels of domain groupings evident: primary domains at scales of the order of 10 nm; domain bundles of the order of 100 nm and groups of bundles at micron length scales. 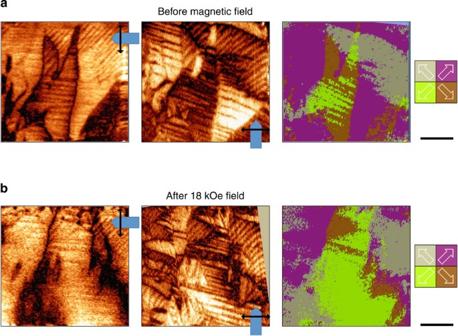Figure 2: Ferroelectric domain configurations changing dramatically with an applied magnetic field. Lateral piezoresponse force microscopy (LPFM) images, before (a) and after (b) the application of a 18-kOe magnetic field, show obvious changes in ferroelectric domain states. In both (a,b) the same region of the PZTFT single-crystal lamella has been scanned. In each case, the left and middle panels are amplitude images, showing variations in the local in-plane piezoelectric activity, with the cantilever orientation in each scan given by the blue schematic tip shape. The directions of tip distortion contributing to the amplitude images are given by the black arrows superposed onto the schematic cantilevers. Domains or packets of domains are clearly distinguished. The right panels are simple in-plane vector maps of the local polarization direction, inferred from the phase signal associated with the amplitude images presented in the middle and left panels. Polar directions are assigned to one of four quadrant directions (grey: left and up; lime green: left and down; purple: right and up; brown: right and down). The magnetic field has caused obvious growth in the domains with polar orientations represented by the lime green colour. Scale bar, 2 μm. Figure 2: Ferroelectric domain configurations changing dramatically with an applied magnetic field. Lateral piezoresponse force microscopy (LPFM) images, before ( a ) and after ( b ) the application of a 18-kOe magnetic field, show obvious changes in ferroelectric domain states. In both ( a , b ) the same region of the PZTFT single-crystal lamella has been scanned. In each case, the left and middle panels are amplitude images, showing variations in the local in-plane piezoelectric activity, with the cantilever orientation in each scan given by the blue schematic tip shape. The directions of tip distortion contributing to the amplitude images are given by the black arrows superposed onto the schematic cantilevers. Domains or packets of domains are clearly distinguished. The right panels are simple in-plane vector maps of the local polarization direction, inferred from the phase signal associated with the amplitude images presented in the middle and left panels. Polar directions are assigned to one of four quadrant directions (grey: left and up; lime green: left and down; purple: right and up; brown: right and down). The magnetic field has caused obvious growth in the domains with polar orientations represented by the lime green colour. Scale bar, 2 μm. Full size image Vertical mode PFM (VPFM) signals were weak, with significant noise contributions, and so different domain orientations have only been interpreted in terms of the in-plane components of their piezoelectric response, using lateral-mode PFM (although VPFM data are explicitly presented in Supplementary information , Supplementary Fig. S1 ). Phase information from such scans indicates the direction (but not the magnitude) of the component of polarization perpendicular to the cantilever axis; by obtaining phase maps for two orthogonal sample orientations, local in-plane polar directions could be assigned into one of four groups: left-up; left-down; right-up and right-down. A kind of domain map (simplified in-plane vector PFM) was hence created, as shown in Fig. 2a right panel. Switching ferroelectric domains with a magnetic field In Fig. 2b , the same region of the PZTFT lamella has been imaged again (in the same orientations as Fig. 2a ), but after the application and removal of a 18 kOe magnetic field, oriented parallel to the lamellar surface. Clearly, dramatic changes in the ferroelectric domain configuration have been induced, best seen in the simplified in-plane vector PFM map in the right panel. Explicit coupling between the applied magnetic field and the resulting ferroelectric domain states is therefore evident. Unfortunately, imaging after exposure to intermediate magnetic fields (below and approaching 18 kOe) did not show significant predictable progressive developments in the domain configuration in this sample (see Supplementary Fig. S2 ). Nevertheless, the possibility of ferroelectric switching using a magnetic field at room temperature has been successfully demonstrated. Not all of the domains had changed after the magnetic field had been applied, but this is in keeping with work by Ponomarev et al . [33] on Tb 2 (MnO 4 ) 3 . Indeed, Hur et al . [5] point out that the complete reorientation of ferroelectric domains by a magnetic field is rarely seen. Hence, our observation of dramatic changes in the overall ferroelectric domain state, even though largely irreversible and stochastic in nature, is still worthy of note. In Fig. 3a(i) , we present LPFM phase information from a region of a different PZTFT single-crystal lamella, after a magnetic field of 3 kOe has been applied perpendicular to the imaged surface and then removed before imaging. Different domains, with in-phase and anti-phase responses, are represented by the blue and red colours. The sense of the magnetic field was subsequently reversed and distinct changes in the phase image, Fig. 3a(ii) , resulted: ferroelectric domains with orientations yielding red phase contrast contracted, while those mapped by blue phase expanded. When the magnetic field was again applied in the original sense, changes in the domain distribution were partially reversed, Fig. 3a(iii) (see also Supplementary Fig. S3 ). 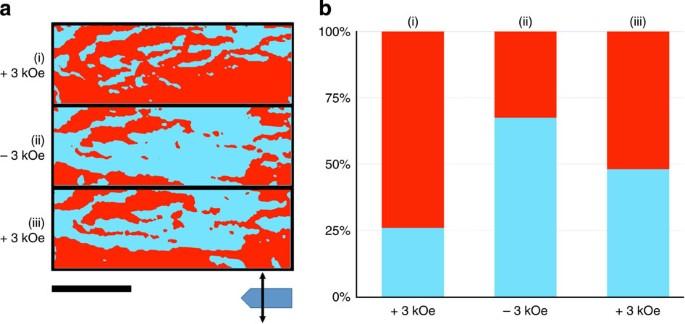Figure 3: Modest magnetic fields induce partially reversible changes in ferroelectric domains. Phase images from lateral piezoresponse force microscopy (LPFM) change depending on the orientation of the magnetic field applied to the PZTFT lamella. Both the images in (a) and the area histograms of different phase colours (b) illustrate that 3 kOe applied in a nominally positive direction, perpendicular to the lamellar surface, favours the growth of polarization directions indicated by red contrast. When applied in a nominally negative direction, these regions contract. Scale bar, 2 μm. Figure 3b summarizes the extent to which magnetically-induced ferroelectric domain changes could be reversed by changing the orientation of the applied magnetic field. Although the changes illustrated in Fig. 3 are not as dramatic as those seen in Fig. 2 , the partial reversibility of the magnetoelectric coupling is an important observation. Definitive equivalent observations could not be made from VPFM ( Supplementary Fig. S4 ) owing to low signal-to-noise in the response. Figure 3: Modest magnetic fields induce partially reversible changes in ferroelectric domains. Phase images from lateral piezoresponse force microscopy (LPFM) change depending on the orientation of the magnetic field applied to the PZTFT lamella. Both the images in ( a ) and the area histograms of different phase colours ( b ) illustrate that 3 kOe applied in a nominally positive direction, perpendicular to the lamellar surface, favours the growth of polarization directions indicated by red contrast. When applied in a nominally negative direction, these regions contract. Scale bar, 2 μm. Full size image Increasing the magnetic field beyond 3 kOe perpendicular to the lamellar surface could increase the degree of ferroelectric domain switching further, but changes became progressively more modest ( Supplementary Fig. S2 ). The PFM mapping techniques used herein have a spatial resolution of the order of tens of nanometres and therefore cannot resolve the nature of any magnetic field-induced microstructural changes at the scale of the finest domain structures imaged in Fig. 1 . Hence, TEM imaging of PZTFT lamellae before and after the application of a magnetic field (3 kOe perpendicular to the lamella surface) was performed ( Fig. 4 ). As can be seen in Fig. 4 , very fine-scale stripe domains appear to coarsen and adopt a labyrinthine structure after the magnetic field has been applied. Whatever the nature of the magnetoelectric coupling, it can clearly affect domain configurations across all length scales. 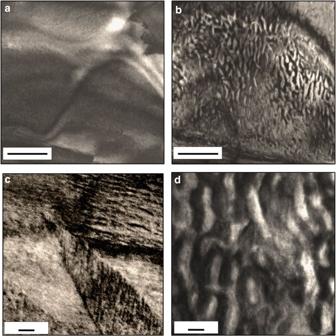Figure 4: Transmission electron microscopy shows distinct changes in domain microstructure induced by magnetic fields. The same region of the sample was imaged (dark field 1–10pcreflection; zone axis <110>pc) before (a) and after (b) the application of a magnetic field of 3 kOe perpendicular to the sample surface. The region imaged in (a) was characterized by bundles of fine-scale domains (c), commensurate withFig. 1. However, quite dramatic changes to coarser ‘labyrinthine’ or ‘maze’ domains, (b,d), were found after exposure to the magnetic field. In (a,b) scale bar, 500 nm; in (c,d) scale bar, 50 nm. Figure 4: Transmission electron microscopy shows distinct changes in domain microstructure induced by magnetic fields. The same region of the sample was imaged (dark field 1–10 pc reflection; zone axis <110> pc ) before ( a ) and after ( b ) the application of a magnetic field of 3 kOe perpendicular to the sample surface. The region imaged in ( a ) was characterized by bundles of fine-scale domains ( c ), commensurate with Fig. 1 . However, quite dramatic changes to coarser ‘labyrinthine’ or ‘maze’ domains, ( b , d ), were found after exposure to the magnetic field. In ( a,b ) scale bar, 500 nm; in ( c , d ) scale bar, 50 nm. Full size image A key element in the characterization of magnetoelectric behaviour involves the determination of a second rank coupling tensor ( α ij ), that describes the rate of change of polarization with respect to the applied magnetic field [1] (for the direct magnetoelectric effect), or alternatively the rate of change of the magnetization with respect to the applied electric field (for the indirect effect) [34] , [35] . Usually, the individual coefficients in the tensor are not explicitly evaluated and instead effective scalar coefficients are stated. For single-phase multiferroics, coupling coefficients are typically of the order of 10 −10 sm −1 (refs 5 , 14 , 27 , 36 ), while for heterostructures values increase to of the order of 10 −6 to 10 −8 sm −1 (refs 14 , 16 , 23 , 27 , 29 , 35 , 37 , 38 , 39 ). To determine an order of magnitude estimate for the effective magnetoelectric coupling coefficient in the PZTFT lamellae investigated in this work, we firstly assume that the magnetic field of 3 kOe has induced ferroelectric domain wall motion comparable to that seen at the coercive electric field in conventional electric field-induced ferroelectric switching. Assuming linear magnetoelectric coupling and linear dielectric behaviour, the formula presented by Eerenstein et al . [39] : (where P is the vector polarisation developed, H is the magnetic field vector and α ij is the linear magnetoelectric coupling tensor) can be re-expressed as: ( ε is the permittivity). At the point at which significant domain movement occurs, an approximate statement: can be made. ε and E coercive (the coercive electrical field) for this material have been determined from Sanchez et al . [24] . Taking H critical as 3 kOe, we hence calculate α 13 eff to be ~5.5 × 10 −8 sm −1 . Another estimate of α 13 eff can be obtained by direct analysis of the data presented in Fig. 3 . If the net electrical displacement in the region imaged in Fig. 3a is taken to be proportional to the difference between the populations of domains with opposite lateral polarisation components (area fraction of red minus area fraction of blue), then the change in this relative domain fraction, as a function of the change in the magnetic field applied, can be determined. For the change in field of 6 kOe (+3 kOe changing to −3 kOe and vice versa), the average change in polarization was found to be 60% of that of the fully poled state (all domains the same colour). By assuming that the maximum electrical displacement in this fully poled state is of the order of 10 μC cm −2 (ref. 24 ) (see Supplementary Information and Supplementary Fig. S5 for a direct quantitative estimate of the lamellar polarisation), we obtain an effective α 13 eff =1.3 × 10 −7 sm −1 , different from the estimate above by approximately a factor of two. This effective coupling coefficient value is surprisingly large and competes with those found to date in magnetoelectric heterostructures [40] . We stress that the effective coupling coefficient has been expressed in terms of the change in polarization for a given applied magnetic field; however, the coupling behaviour will clearly not be linear (hysteresis in the magnetoelectric response is expected). Thus, our effective coupling coefficient does not adhere to the strict definition for α ij where a linear development in polarization with applied magnetic field is assumed. The mechanism by which coupling occurs can only be speculated over at this stage. However, it may be useful to reiterate several aspects of our observations, which might be relevant and would be suggestive of a strain-mediated coupling mechanism: first, the magnetic fields cause changes in the ferroelastic, and not simply the ferroelectric, domain components of the microstructure; second, although some amount of reversibility in domain reorientation has been observed, often the magnetic fields cause sporadic and unpredictable large changes in domain states, commensurate with a sudden release of elastic energy; third, the order of magnitude of the coupling coefficient is comparable to those found in heterostructures where strain-mediated coupling is deliberately targeted (through selection of piezoelectric-magnetostrictive materials combinations for example Lahtinen et al . [23] ). Although many details still remain unresolved at this stage, enough observations have been made to be confident about several points: that PZTFT is a genuine alternative room temperature multiferroic to BiFeO 3 and that a degree of reversibility in the way in which ferroelectric domains expand and contract under magnetic fields can occur. This latter statement could be important, as reversibility is likely to be highly desirable in proposed future multiferroic devices. Coarse-grained PZTFT ceramics were prepared as stated in Sanchez et al . [24] . We used a FEI 200TEM Focused Ion Beam (FIB) to cut out lamellae (~10 × 7 × 0.15–0.3 μm) from single grains of this bulk ceramic. It is worth noting that while each lamella is a single crystal, lamellae are cut from randomly oriented grains and therefore the crystallographic orientation of the lamellar surface is not controlled. For TEM and STEM, lamellae were lifted free from the bulk, using a sharpened glass needle and micromanipulator, and placed onto holey carbon-coated 3 mm copper grids. Selected area electron diffraction was performed in standard TEM mode using 0.5 μm diameter apertures. EDX analysis was done under STEM with a low-background double-tilt holder and typical probe size diameter of the order of 1 nm. A number of single spectra at different points on the lamellae were taken and the average and standard error in cation concentration determined. For PFM, lamellae were placed onto platinum-coated polished single crystals of MgO. These samples were annealed in air at 600 °C for 1 h causing gallium, that had been implanted as a result of FIB processing, to be expelled onto the lamellar surface. This method was based on previous work by Schilling et al . [41] . Expelled gallium, or gallium oxide, was removed by acid etching (5 min in 2.8 mol l −1 HCl) using a procedure based on work by McGilly et al . [42] . PFM was used to directly map magnetic field-induced changes in ferroelectric domain patterns. The 18 kOe field was applied using electromagnets in a vibrating sample magnetometer and the 3 kOe field using permanent (rare earth) magnets. The PFM system detects different ferroelectric domains by monitoring the mechanical distortion of a flexible cantilever with a sharp tip on the end. The tip is electrically conducting, is in contact with the sample and is used to supply a highly localized alternating electric field. Local electric field-induced sample distortion under the tip leads to a movement of the tip-sample contact point, which in turn distorts the cantilever. The PFM monitors both the amplitude of this physical distortion and whether or not it is in or out-of phase with the applied voltage signal. Although both amplitude and phase give useful information, phase maps often give the most accessible picture of ferroelectric domain distribution, as domains with components of polarisation parallel to the applied field move in-phase with the applied voltage, whereas those with polarisation components opposing the field move out-of-phase. Hence in mapping local in-plane polarization orientation in this study, phase information has often been used. How to cite this article: Evans, D. M. et al . Magnetic switching of ferroelectric domains at room temperature in multiferroic PZTFT. Nat. Commun. 4:1534 doi: 10.1038/ncomms2548 (2013).